Observation of resistively detected hole spin resonance and zero-field pseudo-spin splitting in epitaxial graphene Electronic carriers in graphene show a high carrier mobility at room temperature. Thus, this system is widely viewed as a potential future charge-based high-speed electronic material to complement–or replace–silicon. At the same time, the spin properties of graphene have suggested improved capability for spin-based electronics or spintronics and spin-based quantum computing. As a result, the detection, characterization and transport of spin have become topics of interest in graphene. Here we report a microwave photo-excited transport study of monolayer and trilayer graphene that reveals an unexpectedly strong microwave-induced electrical response and dual microwave-induced resonances in the dc resistance. The results suggest the resistive detection of spin resonance, and provide a measurement of the g -factor, the spin relaxation time and the sub-lattice degeneracy splitting at zero magnetic field. The quantum mechanical spin degree of freedom finds remarkable applications in the areas of quantum computing (QC) and spin-based electronics (spintronics) [1] , [2] , [3] , [4] , [5] , [6] , [7] , [8] . For example, in QC scenarios, particle spin often serves as a quantum bit or qubit [1] , [2] , [3] , [4] , [5] , [6] . In spintronics, the spin serves to endow electronic devices with new functionality as in the giant magneto-resistive read head or the spin-based transistor [7] , [8] . Graphene is a novel two-dimensional system with remarkable properties such as massless Dirac fermions, an anomalous Berry's Phase, a pseudo-spin (valley degeneracy) in addition to spin and half-integral quantum Hall effect [9] , [10] , [11] , [12] . Graphene is also an appealing material for electron-spin QC and spintronics [1] , [4] , [5] , [6] , [7] , [8] , [13] , [14] , [15] , owing to the expected weak spin–orbit interaction and the scarcity of nuclear spin in natural carbon. Because of QC and spintronics, the microwave control and electrical detection of spin have become topics of interest now in graphene nanostructures [1] , [2] , [3] , [4] , [5] , [6] , [7] , [8] , [9] , [10] , [11] , [12] , [13] , [14] , [15] , [16] , [17] , where the small number of spins limits the utility of traditional spin resonance. Here we report the first observation of resistive detection of spin resonance in epitaxial graphene (EG) [9] , [18] , [19] , provide a measurement of the g -factor and the spin relaxation time, and determine the pseudo-spin (valley degeneracy) splitting at zero magnetic field. Such resistive resonance detection can potentially serve to directly characterize the spin properties of Dirac fermions, and also help to determine and tune the valley-degeneracy splitting for spin-based QC [15] . 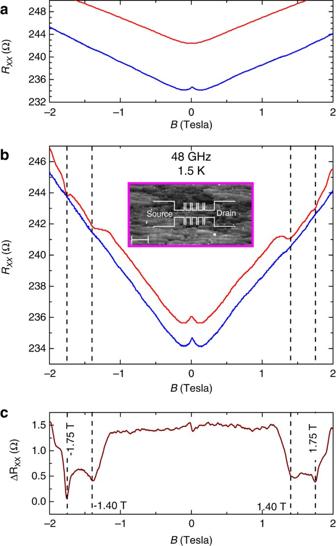Figure 1: Transport in trilayer graphene. (a) The diagonal resistance,Rxx, is shown versus the magnetic field,B, at temperaturesT=90 K, shown in red, andT=1.5 K, shown in blue, for sample 1, in the dark condition, without microwave excitation. The upward displacement of theT=90 K curve with respect to theT=1.5 K curve shows thatRxxincreases with the temperature, that is, dRxx/dT≥0. (b)RxxversusBin the absence of microwave excitation is shown in blue, and under constantF=48 GHz microwave excitation atP=4 mW is shown in red, for sample 1. The photo-excitedRxxtrace shown in red exhibits a uniform upward shift with respect to the darkRxxcurve shown in blue forB<1 T. At higherB, resonant reductions in theRxxare observed in the vicinity ofB=±1.4 and ±1.75 T, where the photo-excitedRxxapproaches the dark value. Inset: an atomic force microscopy image of the EG/SiC surface with the device superimposed upon it. The size scale bar corresponds to 10 μm. (c) The change in the diagonal resistance, ΔRxx, between the photo-excited and dark conditions in panelb, that is, ΔRxx=Rxx(4 mW)−Rxx(dark), is shown versusB. Note the valleys in ΔRxxin the vicinity ofB=±1.40 and ±1.75 T. Trilayer graphene Figure 1a shows the diagonal resistance, R xx , versus the magnetic field, B , for the trilayer EG specimen, sample 1. The blue curve obtained at T =1.5 K in sample 1 shows a cusp in R xx near null magnetic field, that is, weak localization (WL) [20] , [21] , [22] , followed by positive magneto-resistance at B >0.2 T. In Fig. 1a , an increase in T , to T =90 K, results in the red curve, which includes a positive displacement of the R xx versus B trace with respect to the T =1.5 K trace, that is, d R xx /d T >0 at B =0 T, along with the quenching of WL. As WL cannot be observed without inter-valley scattering in monolayer or bilayer graphene [22] , the observed WL is presumed to be an indicator of a non-zero inter-valley matrix element. Figure 1: Transport in trilayer graphene. ( a ) The diagonal resistance, R xx , is shown versus the magnetic field, B , at temperatures T =90 K, shown in red, and T =1.5 K, shown in blue, for sample 1, in the dark condition, without microwave excitation. The upward displacement of the T =90 K curve with respect to the T =1.5 K curve shows that R xx increases with the temperature, that is, d R xx /d T ≥0. ( b ) R xx versus B in the absence of microwave excitation is shown in blue, and under constant F =48 GHz microwave excitation at P =4 mW is shown in red, for sample 1. The photo-excited R xx trace shown in red exhibits a uniform upward shift with respect to the dark R xx curve shown in blue for B <1 T. At higher B , resonant reductions in the R xx are observed in the vicinity of B =±1.4 and ±1.75 T, where the photo-excited R xx approaches the dark value. Inset: an atomic force microscopy image of the EG/SiC surface with the device superimposed upon it. The size scale bar corresponds to 10 μm. ( c ) The change in the diagonal resistance, Δ R xx , between the photo-excited and dark conditions in panel b , that is, Δ R xx = R xx (4 mW)− R xx (dark), is shown versus B . Note the valleys in Δ R xx in the vicinity of B =±1.40 and ±1.75 T. Full size image Figure 1b illustrates the influence of microwave excitation on sample 1 at F =48 GHz. Here, for B <1 T, microwave excitation produces a positive displacement of the photo-excited R xx relative to the blue trace obtained in the absence of photo-excitation, akin to increasing the temperature, cf. Fig. 1a . However, at B >1 T, R xx shows resistance valleys as the photo-excited curve approaches the dark curve, similar to reducing the temperature. To highlight associated resonances, the change in the diagonal resistance, Δ R xx = R xx (4 mW)− R xx (dark), is shown versus B in Fig. 1c . 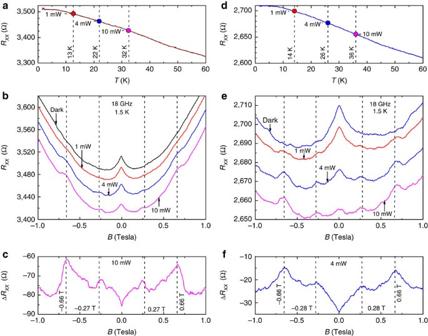Figure 2: Transport in single-layer graphene. Panelsa–cshow some results for sample 2, whereas figsd,fshow representative data for sample 3. (a) Sample 2 shows a decrease in the resistanceRxxwith increasing temperatureT, that is, dRxx/dT≤0, in the absence of a magnetic field, that is,B=0 T. (b) The data traces show a downward shift with increasing microwave power,P, atF=18 GHz, suggestive of microwave-induced carrier heating in the specimen. TheRxxatB=0 T obtained from these traces have been marked as filled circles in panelaabove, which shows theTdependence ofRxx. Apparently,P=10 mW serves to increase the carrier temperature up toT=32 K in sample 2. Microwave-induced resonances appear in the vicinity of the dashed lines with increasingP. (c) ΔRxx=Rxx(10 mW)−Rxx(dark) is shown versus the magnetic field for sample 2. Note the change in ΔRxxdue to spin resonance in the vicinity of the dashed lines atB=±0.66 and ±0.27 T. (d) Sample 3 also shows a decrease in the resistanceRxxwith increasing temperatureT, that is, dRxx/dT≤0, in the absence of a magnetic field, that is,B=0 T. (e) AtF=18 GHz andT=1.5 K,Rxxis shown versusBfor sample 3, at several power levels. TheRxxatB=0 T observed in these data have been marked as filled circles in paneld. (f) This panel shows ΔRxx=Rxx(10 mW)−Rxx(dark) versus the magnetic field for sample 3. Note the change in ΔRxxdue to spin resonance in the vicinity ofB=±0.66 and ±0.28 T. Figure 1c shows two noteworthy features: a high magnetic field resonance at | B |=1.75 T and a low magnetic field feature at | B |=1.4 T. These resonances disappeared upon increasing the bath temperature to T >5 K. Monolayer graphene Figure 2a–c shows the results for sample 2, whereas Fig. 2d–f shows representative data for sample 3. Both sample 2 and sample 3 are monolayer EG specimens. The T dependence of R xx at B =0 T is shown in Fig. 2a for samples 2 and 3, respectively. Unlike sample 1, samples 2 and 3 show a decrease in R xx ( B =0) with increasing temperature, that is, d R xx /d T ≤0. Further, as indicated in Fig. 2b , microwave irradiation of these specimens produces a uniform negative displacement in the R xx traces with increasing power, P . Yet, the effect of microwave excitation (d R xx /d P ≤0 at B =0) is again similar to heating the specimen (d R xx /d T ≤0), cf. Fig. 2a . Thus, the R xx ( B =0) regions from Fig. 2b have been marked as coloured discs in Fig. 2a . Apparently, microwave excitation at P =10 mW serves to increase the carrier temperature up to T =32 K in sample 2, and up to T =36 K in sample 3. At such higher P , the radiation helps to manifest, in addition, resonant R xx peaks in the vicinity of the dashed lines of Fig. 2b , unlike in Fig. 1b , where valleys characterize the resonances in R xx . Yet, in all three specimens, the photo-excited R xx moves towards the dark curve at resonance. Fig. 2c shows resonances at nearly the same | B |, at F =18 GHz, in samples 2 and 3. Figure 2: Transport in single-layer graphene. Panels a – c show some results for sample 2, whereas figs d , f show representative data for sample 3. ( a ) Sample 2 shows a decrease in the resistance R xx with increasing temperature T , that is, d R xx /d T ≤0, in the absence of a magnetic field, that is, B =0 T. ( b ) The data traces show a downward shift with increasing microwave power, P , at F =18 GHz, suggestive of microwave-induced carrier heating in the specimen. The R xx at B =0 T obtained from these traces have been marked as filled circles in panel a above, which shows the T dependence of R xx . Apparently, P =10 mW serves to increase the carrier temperature up to T =32 K in sample 2. Microwave-induced resonances appear in the vicinity of the dashed lines with increasing P . ( c ) Δ R xx = R xx (10 mW)− R xx (dark) is shown versus the magnetic field for sample 2. Note the change in Δ R xx due to spin resonance in the vicinity of the dashed lines at B =±0.66 and ±0.27 T. ( d ) Sample 3 also shows a decrease in the resistance R xx with increasing temperature T , that is, d R xx /d T ≤0, in the absence of a magnetic field, that is, B =0 T. ( e ) At F =18 GHz and T =1.5 K, R xx is shown versus B for sample 3, at several power levels. The R xx at B =0 T observed in these data have been marked as filled circles in panel d . ( f ) This panel shows Δ R xx = R xx (10 mW)− R xx (dark) versus the magnetic field for sample 3. 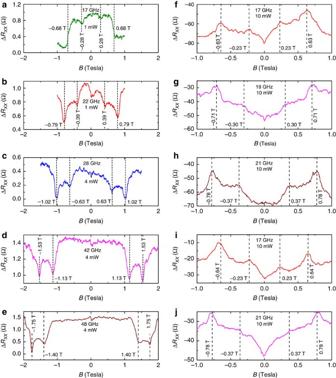Figure 3: Frequency evolution of microwave-induced resonances. (a–e) For sample 1, the photo-induced change in the diagonal resistance, ΔRxx, is plotted versusBfor (a) 17 GHz, (b) 22 GHz, (c) 28 GHz, (d) 42 GHz and (e) 48 GHz. Note the uniform shift in the resonances, indicated by dashed lines, to higherBwith increasingF. Here, the resonances are characterized by ΔRxxminima. (f–h): For sample 2, the photo-induced change in the diagonal resistance, ΔRxx, is plotted versusBfor (f) 17 GHz, (g) 19 GHz and (h) 21 GHz. Note the shift in the resonances, indicated by dashed lines, to higherBwith increasingF. Here, the resonances are characterized by resistance maxima. (i,j) For sample 3, the photo-induced change in the diagonal resistance, ΔRxx, is plotted versusBfor (i) 17 GHz and (j) 21 GHz. Note the shift in the resonances, indicated by dashed lines, to higherBwith increasingF. Note the change in Δ R xx due to spin resonance in the vicinity of B =±0.66 and ±0.28 T. Full size image Spin resonance evolution Figure 3 illustrates the frequency evolution of the Δ R xx resonances for all three specimens. Here, Fig. 3a–e illustrates the results for sample 1, Fig. 3f–h exhibits the data for sample 2 and Fig. 3i shows some results for sample 3. Note the shift of resonances to higher B with increasing F . Figure 3: Frequency evolution of microwave-induced resonances. ( a – e ) For sample 1, the photo-induced change in the diagonal resistance, Δ R xx , is plotted versus B for ( a ) 17 GHz, ( b ) 22 GHz, ( c ) 28 GHz, ( d ) 42 GHz and ( e ) 48 GHz. Note the uniform shift in the resonances, indicated by dashed lines, to higher B with increasing F . Here, the resonances are characterized by Δ R xx minima. ( f – h ): For sample 2, the photo-induced change in the diagonal resistance, Δ R xx , is plotted versus B for ( f ) 17 GHz, ( g ) 19 GHz and ( h ) 21 GHz. Note the shift in the resonances, indicated by dashed lines, to higher B with increasing F . Here, the resonances are characterized by resistance maxima. ( i , j ) For sample 3, the photo-induced change in the diagonal resistance, Δ R xx , is plotted versus B for ( i ) 17 GHz and ( j ) 21 GHz. Note the shift in the resonances, indicated by dashed lines, to higher B with increasing F . 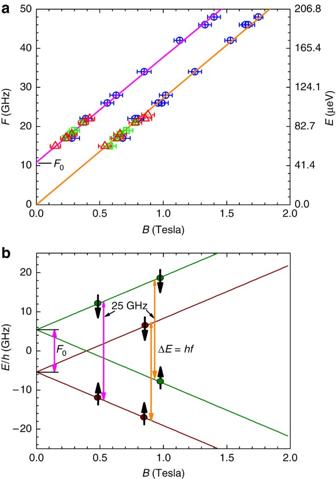Figure 4: Relation between the resonance magnetic fields and the microwave frequency or energy. (a) This plot shows that the highB-field resonance found inFig. 3follows a linear fit, indicated by the gold line, asF(GHz)=27.2B(T) with an intercept at the origin. The lowB-field resonance found inFig. 3, indicated by the magenta line, follows a linear fit asF(GHz)=10.76+26.9B(T) with a non-zero intercept,F0=10.8 GHz. Here, the lines indicate the fits, while the symbols show the data points. The circles correspond to the data for sample 1, the squares correspond to the data for sample 2 and the triangles correspond to the data for sample 3. (b) The observed experimental results appear to be consistent with spin resonance and zero-field pseudo-spin (valley-degeneracy) splitting enhanced spin resonance. A fourfold degeneracy is lifted in the absence of a magnetic field to produce a pair of spin degenerate levels (doublets) separated byE/h=F0. Zeeman splitting then lifts the spin degeneracy of the upper and lower doublets. Microwave photo-excitation induces spin-flip transitions between the spin levels of the lower- or upper doublet, as shown by the gold lines. Such transitions require vanishing photon energy in theB→0 limit. On the other hand, the transition shown in magenta requires non-vanishing photon energy in the limit ofB→0. Full size image Figure 4a presents a plot of the microwave frequency, F , versus the resonance magnetic fields, B , extracted from Fig. 3 . Figure 4a shows that the resonance B values for the three specimens collapse onto two lines: a gold-coloured line in Fig. 4a , which represents the high B -field resonances of Fig. 3 , shows a linear increase as F (GHz)=27.2 B ( T ), with the ordinate intercept at the origin. Another line shown in magenta in Fig. 4a , which represents the low- B resonances of Fig. 3 , shows a linear increase as F (GHz)=10.76+26.9 B ( T ), with a non-zero intercept, F 0 =10.76 GHz. In such a plot, spin resonance for an electron with g -factor g e =2.0023 would follow: F (GHz)=28.01 B (T). Thus, the observed slopes, d F /d B =26.9±0.4 GHz T −1 (d F /d B =27.2±0.2 GHz T −1 ) for the low (high) field resonance correspond to spin resonances with g // =1.92±0.028 ( g // =1.94±0.014). Figure 4: Relation between the resonance magnetic fields and the microwave frequency or energy. ( a ) This plot shows that the high B -field resonance found in Fig. 3 follows a linear fit, indicated by the gold line, as F (GHz)=27.2 B ( T ) with an intercept at the origin. The low B -field resonance found in Fig. 3 , indicated by the magenta line, follows a linear fit as F (GHz)=10.76+26.9 B ( T ) with a non-zero intercept, F 0 =10.8 GHz. Here, the lines indicate the fits, while the symbols show the data points. The circles correspond to the data for sample 1, the squares correspond to the data for sample 2 and the triangles correspond to the data for sample 3. ( b ) The observed experimental results appear to be consistent with spin resonance and zero-field pseudo-spin (valley-degeneracy) splitting enhanced spin resonance. A fourfold degeneracy is lifted in the absence of a magnetic field to produce a pair of spin degenerate levels (doublets) separated by E / h = F 0 . Zeeman splitting then lifts the spin degeneracy of the upper and lower doublets. Microwave photo-excitation induces spin-flip transitions between the spin levels of the lower- or upper doublet, as shown by the gold lines. Such transitions require vanishing photon energy in the B →0 limit. On the other hand, the transition shown in magenta requires non-vanishing photon energy in the limit of B →0. Full size image The g -factors measured here are comparable to the g-values obtained from traditional ESR studies of graphite, which have indicated that the g -factor for c -axis, , increases from 2.05 at 300 K to 2.15 at 77 K, while, at T =300 K, the g -factor for c -axis, =2.003 (refs 23 , 24 ). In graphite, the g -factor depends upon the orientation of the B field, the temperature, the location of the Fermi level and the sign of the charge carriers, with opposite g -factor shifts, Δ g , from g e , for electrons and holes [23] , [24] , [25] . The negative Δ g and reduced g // observed here relative to g e are consistent with expectation for holes. From these data, we also estimate a resonance half-width Δ B ≈0.05 T, which corresponds to a spin relaxation time τ s = h /(4 π Δ E )=6 × 10 −11 s. The spin relaxation time has been a topic of great interest in graphene. Spin relaxation [26] has been experimentally studied in monolayer and bilayer exfoliated graphene on SiO 2 /Si (refs 27 , 28 , 29 , 30 , 31 , 32 , 33 , 34 ) and, more recently, on EG [35] , [36] using spin valve devices, and possible mechanisms involved in spin relaxation have been examined by theory [37] , [38] , [39] . For monolayer exfoliated graphene, observed spin relaxation times generally fall in the range of 40–150 ps (refs 28 , 30 , 31 , 34 ), while exfoliated bilayer graphene shows spin relaxation times as long as 2–6 ns (refs 32 , 33 ). The observed shorter-than-expected spin lifetime in exfoliated monolayer graphene has been attributed to extrinsic mechanisms based on impurity adatoms [37] , charged impurities and phonons from the substrate [38] , spin–orbit coupling due to ripples in graphene [39] , and so on. Note that the τ s reported here for C -face EG is comparable to previous reports of the spin relaxation time for monolayer exfoliated graphene on SiO 2 /Si. The spin-diffusion length here is λ s =( Dτ s ) 1/2 =1.4 μm (ref. 13 ), while the Hall bar width, w =4 μm. Here, D is the diffusion constant. In such a situation, edges could be having a role in spin relaxation, given that edges in graphene can be magnetically active [12] , and the electrical contacts include gold, a heavy element. Thus, there could be additional avenues for spin relaxation in the small specimen, in addition to the other above-mentioned mechanisms [37] , [38] , [39] . Finally, inhomogeneities could serve to broaden the resonance linewidth and help to produce an apparently reduced spin relaxation time. The observation of similar double resonances in monolayer and trilayer graphene can be viewed as a consequence of rotational (non-AB) layer stacking in EG, which makes it possible even for multilayer EG to show the same electronic properties as isolated graphene [18] . Note also that sub-lattice or pseudo-spin degeneracy lifting is known to occur at high B in graphene [40] , [41] , [42] . For example, the progression of quantum Hall effect from the R xy =[4( N +1/2)] −1 h / e 2 sequence [10] , [11] , [43] , to observations of σ xy increases in steps of e 2 / h (ref. 40 ), reflects the lifting of both the spin- and pseudo-spin degeneracy. In addition, a non-linear interaction-enhanced valley-degeneracy splitting has been reported from a scanning tunnelling spectroscopy study [42] . Finally, the manifestation of WL, which is observable in Figs 1 and 2 , is an indicator of inter-valley coupling in these specimens [22] . As sub-lattice degeneracy splitting is not unexpected owing to the above, the observed F 0 =10.76 GHz is attributed to a zero magnetic field pseudo-spin (sub-lattice degeneracy) splitting of Δ 0 = hF 0 =44.4 μeV. A provisonal interpretation of the F versus B plot of Fig. 4a is provided in Fig. 4b . Chiral eigenstates and linear energy-wavevector dispersion characterize carriers in graphene. The application of a B field nominally produces fourfold, valley- and spin-degenerate Landau levels characterized by E N =± ν F (2 eħBN ) 1/2 , where N =0, 1, 2…, e is the electron charge, ν F is the Fermi velocity and ħ is the reduced Planck's constant. We imagine the fourfold degeneracy being lifted by hF 0 even at B =0, to produce energy doublets as E N ′ = E N ± hF 0 /2. Then, owing to the Zeeman effect, associated Landau levels show a further splitting of the spin degeneracy as E N ″ = E N ′ ± gμB /2. Observed microwave-induced transitions occur within the highest occupied Landau level in the vicinity of the Fermi level. As E N >> hF 0 /2 and gμB /2, we remove the E N term and plot E / h =( E N ″ − E N )/ h in Fig. 4b . Here, microwave photo-excitation induces spin-flip transitions, shown in gold, of unpaired carriers between the spin levels of the lower or the upper doublet. Such transitions require vanishing photon energy in the limit of vanishing B . In contrast, a transition between the lower spin ('up') level of the lower doublet and the higher spin ('down') level of the upper doublet requires additional energy hF 0 , and such a transition, shown in magenta, exhibits non-vanishing photon energy in the B →0 limit. Thus, the F versus B plot appears consistent with spin resonance and a zero-field pseudo-spin (valley degeneracy) splitting enhanced spin resonance. In summary, we have realized the resistive detection of spin resonance in EG, provided a measurement of the g -factor and the spin relaxation time, and identified—and measured—a pseudo-spin (valley degeneracy) splitting in the absence of a magnetic field. Such resistive resonance detection can potentially serve to directly characterize the spin properties of Dirac fermions, and also help to determine—and tune—the valley-degeneracy splitting for spin-based QC. Graphene samples EG was realized by the thermal decomposition of insulating 4H silicon carbide (SiC) [18] . The EG specimens were characterized by ellipsometry and the extracted layer thickness was converted to the number of layers at the rate of 0.335 nm per layer. The C -face of the EG/SiC chip was processed by e-beam lithography into micron-sized Hall bars with Pd/Au contacts. Measurements are reported here for three Hall bar specimens labelled 1, 2 and 3. Sample 1 is nominally trilayer graphene, while samples 2 and 3 are monolayer graphene. The samples are p-type, with a hole concentration, p ≈10 13 cm −2 , and a carrier mobility μ ≈10 3 cm 2 V −1 s −1 . Measurement configuration Typically, an EG Hall bar specimen was mounted at the end of a long straight section of WR-62 rectangular microwave waveguide. The waveguide with sample was inserted into the bore of a superconducting solenoid, immersed in pumped liquid Helium and irradiated with microwaves over the frequency range 10≤ F ≤50 GHz, at a source power 0.1≤ P ≤10 mW, as in the usual microwave-irradiated transport experiment [44] . Here, the applied external magnetic field was oriented along the solenoid and waveguide axis, as a probe-coupled antenna launcher excited the Transverse Electric (TE-10) mode in the waveguide. Thus, the microwave electric field was oriented perpendicular to the applied external magnetic field. The microwave magnetic field lines formed closed loops, with components in the transverse and axial directions of the waveguide. How to cite this article: Mani, R.G. et al . Observation of resistively detected hole spin resonance and zero-field pseudo-spin splitting in graphene. Nat. Commun. 3:996 doi: 10.1038/ncomms1986 (2012).